Steller’s sea cow uncertain history illustrates importance of ecological context when interpreting demographic histories from genomes 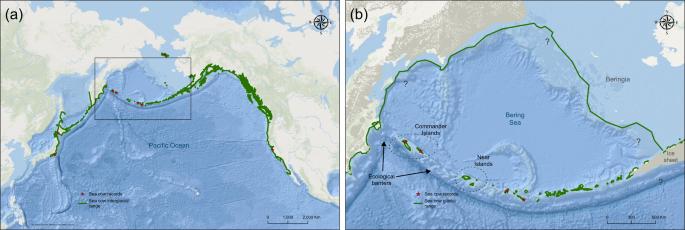Fig. 1: Steller’s sea cow (Hydrodamalis gigas) range reconstructions. (a) Interglacial range. (b) Range during glacial maxima. The Commander Islands have always been physically isolated by deep channels - even during lowest sea levels - that likely constituted ecological barriers, or biogeographic breaks, for sea cows. Different lines of evidence (e.g., absence of echolocation or other navigational apparatus13; limited ability to submerge9; exclusive seaweed diet10) converge to a strictly coastal, ‘linear elongated’ distribution along kelp-dominated shorelines, a range that coincided with that of the sea otter,Enhydra lutris13. Sea cow range reconstructions were based on: (1) review of existing sea cow records (see Dataset); (2) bioindicators of sea cow habitat (i.e., kelp forests, sea otter historical ranges14); (3) southern extent of winter drift ice and year-round kelp habitat;15,16and (4) the estimated shoreline of Beringia and Bering Sea islands during the Last Glacial Maximum12. ‘Sea cow records’ (red stars) refer to undisputed records only. Question marks refer to uncertainties related to sea ice extent along the shoreline of Beringia during glacial times. Map background image source and license: Maps were created using ArcGIS Online basemap ‘World Ocean Base’ (Esri, GEBCO, DeLorne, NaturalVue) and using ArcGIS® software by Esri. ArcGIS® and ArcMap™ are the intellectual property of Esri and are used herein under license. Copyright © Esri. All rights reserved. For more information about Esri® software, please visitwww.esri.com. Further information on research design is available in the Nature Research Reporting Summary linked to this article.